A common variant at 8q24.21 is associated with renal cell cancer Renal cell carcinoma (RCC) represents between 80 and 90% of kidney cancers. Previous genome-wide association studies of RCC have identified five variants conferring risk of the disease. Here we report the results from a discovery RCC genome-wide association study and replication analysis, including a total of 2,411 patients and 71,497 controls. One variant, rs35252396[CG] located at 8q24.21, is significantly associated with RCC after combining discovery and replication results (OR=1.27, P combined =5.4 × 10 −11 ) and has an average risk allele frequency in controls of 46%. rs35252396[CG] does not have any strongly correlated variants in the genome and is located within a region predicted to have regulatory functions in several cell lines, including six originating from the kidney. This is the first RCC variant reported at 8q24.21 and it is largely independent ( r 2 ≤0.02) of the numerous previously reported cancer risk variants at this locus. Established risk factors for renal cell carcinoma (RCC) are smoking, obesity and hypertension. Risk of RCC has also been shown to have a strong genetic component, both in rare hereditary syndromes as well as in the general population [1] , [2] , [3] . Rare, high-penetrance mutations accounting for syndromic RCC have been found in several genes, including VHL , MET , FLCN and FH [4] . Genome-wide association studies (GWAS) have reported five sporadic RCC susceptibility loci [5] , [6] , [7] . However, in combination, these risk variants account for only a small fraction of the approximately twofold greater than the average risk of RCC in first-degree relatives of RCC patients [1] , [2] . Hence, it is likely to be that several more such variants exist. Here we report results from a RCC GWAS study of Icelandic subjects. Our initial scan and replication study yields a common variant at 8q24.21 associated with the disease. This variant does not have any strongly correlated variants in the genome and is located within a region predicted to have regulatory functions in several cell lines, including six originating from the kidney. GWAS data and imputation in Icelandic samples To search for RCC risk variants, we analysed data generated by the ongoing whole-genome sequencing project at deCODE genetics. The variants discovered in the sequencing phase are propagated into chip-genotyped individuals and into relatives of chip-genotyped individuals, making use of the extensive genealogical information available in Iceland and previously reported phasing and imputation methods [8] . At the time that the association analysis in our study was performed, 2,230 Icelanders had been sequenced to at least tenfold coverage. The ~38.5 million variants discovered through whole-genome sequencing were imputed into 95,085 Icelanders who had all been genotyped using commercial Illumina chips, as well as into 296,526 Icelanders without direct chip genotypes but with family-based imputation genotype information [8] , [9] (see Methods). Our list of RCC patients contains 1,667 individuals diagnosed from 1955 until end of 2011, based on the nationwide Icelandic Cancer Registry (ICR; http://www.krabbameinsskra.is/indexen.jsp?icd=C64 ). The GWAS association results presented here are based on the imputation of 575 Icelandic patients who had been genotyped using one of the commercial Illumina single-nucleotide polymorphism (SNP) chips, as well as on 930 Icelandic patients who had at least partial genotype data based on family-based imputation. As controls we used imputed data from 67,725 individuals (25,875 had variants imputed based on chip genotypes and 41,850 had variants imputed with family-based methods) not diagnosed with RCC according to the nationwide ICR. In the present RCC GWAS, only variants with an imputed genotype information measure value >0.9 were used (for a Q – Q plot, see Fig. 1 ). 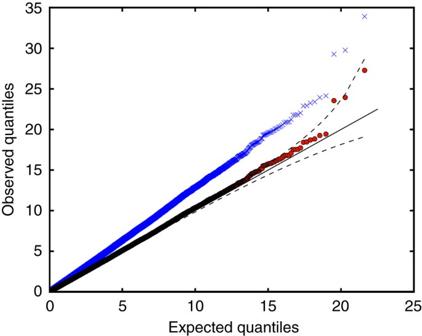Figure 1:AQ–Qplot of the RCC GWAS results. The plot shows the uncorrected (blue crosses) and corrected (using the method of genomic control; red circles)χ2-statistics from the RCC GWAS. This data set consists ofχ2-values for 300,843 SNPs present on the Illumina chips used to genotype the Icelandic study samples. The broken lines are boundaries of the theoretical 95% point-wise confidence band (assuming independentχ2-variables). The solid black equiangular line is displayed for reference purposes. Figure 1: A Q – Q plot of the RCC GWAS results. The plot shows the uncorrected (blue crosses) and corrected (using the method of genomic control; red circles) χ 2 -statistics from the RCC GWAS. This data set consists of χ 2 -values for 300,843 SNPs present on the Illumina chips used to genotype the Icelandic study samples. The broken lines are boundaries of the theoretical 95% point-wise confidence band (assuming independent χ 2 -variables). The solid black equiangular line is displayed for reference purposes. Full size image Genetic association with RCC According to our RCC GWAS data set, association results for four [5] , [6] of the five previously reported GWAS-identified RCC susceptibility variants are confirmed ( P between 0.011 and 3.0 × 10 −4 for SNPs on 2p12, 11q13.3, 12p11.23 and 12q24.31 ( Table 1 ) generated from logistic regression analysis). Logistic regression is used throughout to test for association between SNPs and disease. Results for the fifth variant, located on 2q22.3, are nonsignificant but the effect is in the same direction as originally reported [7] ( P =0.51, odds ratio (OR)=1.10). Table 1 Association results for the Icelandic study population and variants at previously reported RCC GWAS loci. Full size table The most significant variant associated with RCC in our GWAS was rs35252396[CG] located at 8q24.21 (OR=1.30, P =1.8 × 10 −7 ). This variant is a two base pair substitution, and according to NCBI-dbSNP it is classified as a multiple nucleotide variation with alleles of common length >1, but it has also been annotated as two consecutive single-nucleotide variations: rs6470588(A/C) and rs6470589(C/G). Notably, rs6470588 is in both the HapMap and the 1,000 Genome Project imputation reference panels and it is also on most versions of the widely used Illumina genome-wide genotyping chips. No significant difference was observed when the Icelandic patients were stratified according to gender, age at diagnosis or aggressiveness of the disease at the time of diagnosis (that is, comparison of patients with stage T3 or higher, node-positive or metastatic disease with the group of patients with stage T2 or lower). rs35252396 is located at 8q24.21 where numerous independent variants have been shown to confer risk of both haematological and solid cancers but have not previously shown to confer risk of RCC. rs35252396 is located 136 Kb telomeric to MYC , ~13.5 Kb upstream of the non-protein coding gene PVT1 (according to the gene’s RefSeq NR_003367.2 coordinates; Fig. 2 ). However, the PVT1 locus is complex and several mRNA splice variants have been identified, some of which have a transcription initiation site centromeric to rs35252396 (the PVT1 locus is reviewed in Huppi et al. [10] ). Of the previously published cancer risk SNPs at 8q24, the one located closest to rs35252396 is the urinary bladder cancer risk SNP rs9642880 (ref. 11 ). The correlation between these two variants is very weak ( r 2 =0.015), and the correlations between the RCC risk variant and other published cancer risk variants at 8q24 are even weaker ( Supplementary Table S1 ). No significant association was observed in our analysis between RCC and any of the previously reported cancer risk variants at 8q24. 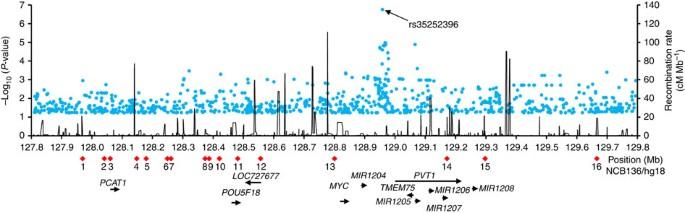Figure 2: Schematic view of the 8q24 region containing rs35252396 and several other disease risk variants. Shown are imputed association results (blue circles) for variants withP<0.05 in the Icelandic RCC GWAS and located on 8q24.21 between 127.8 Mb and 129.8 Mb (Build 36). Logistic regression was used to test for association between SNPs and phenotype. The red diamonds below thexaxis denote the previously reported disease risk variants at 8q24 in populations of European descent (1, rs12543663 (ref.29); 2, rs10086908 (refs29,30); 3, rs1016343 (ref.29); 4, rs13252298 (ref.29); 5, rs16901979 (ref.31); 6, rs188140481 (ref.32); 7, rs2456449 (ref.33); 8, rs16902094 (ref.34); 9, rs445114 (ref.34)/rs620861 (refs29,35); 10, rs6983267 (ref.36); 11, rs1447295 (ref.37); 12, rs13281615 (ref.38); 13, rs9642880 (ref.11); 14, rs2648875 (ref.12); 15, rs2019960 (ref.39); 16, rs10088218 (ref.40); see alsoSupplementary Table S1) and the black arrows represent genes in the region according to the RefSeq database (the size ofPVT1is according to RefSeq NR_003367.2). The black traces represent the recombination rate based on results from the Utah residents of Northern and Western European ancestry (CEU) HapMap population. Figure 2: Schematic view of the 8q24 region containing rs35252396 and several other disease risk variants. Shown are imputed association results (blue circles) for variants with P <0.05 in the Icelandic RCC GWAS and located on 8q24.21 between 127.8 Mb and 129.8 Mb (Build 36). Logistic regression was used to test for association between SNPs and phenotype. The red diamonds below the x axis denote the previously reported disease risk variants at 8q24 in populations of European descent (1, rs12543663 (ref. 29 ); 2, rs10086908 (refs 29 , 30 ); 3, rs1016343 (ref. 29 ); 4, rs13252298 (ref. 29 ); 5, rs16901979 (ref. 31 ); 6, rs188140481 (ref. 32 ); 7, rs2456449 (ref. 33 ); 8, rs16902094 (ref. 34 ); 9, rs445114 (ref. 34 )/rs620861 (refs 29 , 35 ); 10, rs6983267 (ref. 36 ); 11, rs1447295 (ref. 37 ); 12, rs13281615 (ref. 38 ); 13, rs9642880 (ref. 11 ); 14, rs2648875 (ref. 12 ); 15, rs2019960 (ref. 39 ); 16, rs10088218 (ref. 40 ); see also Supplementary Table S1 ) and the black arrows represent genes in the region according to the RefSeq database (the size of PVT1 is according to RefSeq NR_003367.2). The black traces represent the recombination rate based on results from the Utah residents of Northern and Western European ancestry (CEU) HapMap population. Full size image In addition to cancer risk variants, 8q24 has been reported to contain variants, located intragenic in PVT1 , associated with end-stage renal disease in type 2 diabetics [12] . The strongest variant (rs2648875) is very weakly correlated with the RCC variant reported here ( r 2 =0.009) and rs2648875 is not associated with RCC in our analysis. We proceeded to validate the Icelandic RCC association results for rs35252396 on 8q24 by genotyping it by using a single-track assay in two RCC study groups of European descent coming from the Netherlands and Spain. The results of the two study groups showed significant association ( P =5.9 × 10 −5 ), and combining them with the results from Iceland gave an estimated OR of 1.27 for rs35252396[CG] ( P comb =5.4 × 10 −11 ; Table 2 ). A test of heterogeneity of the ORs of all three study groups showed no significant difference ( P het =0.67; Table 2 ). We also genotyped rs35252396 in 1,678 Icelanders, using a single-track assay, to confirm the imputed Icelandic results. The correlation between the imputed and measured genotypes was high ( r =0.98). As a final confirmation, we Sanger sequenced 395 samples from the three study populations and compared the results with the single-variant genotyping results for rs35252396. The correlation between these two data sets was also high ( r =0.97). Table 2 Summary association results for rs35252396 and RCC. Full size table When examining the fit of the genotypes of rs35252396 to the different models of inheritance, using only results generated by single-variant assay genotyping from all three study populations, the multiplicative model provided an adequate fit. Because of the high frequency of the risk allele of rs35252396, homozygous carriers are ~21% of the general population and they have an estimated OR of 1.48 when compared with non-carriers ( Table 3 ). Table 3 Genotypic association results for rs35252396. Full size table Interestingly, rs35252396 has no strongly correlated ( r 2 >0.5) variants, according to our analysis of the genomes of 2,230 whole-genome-sequenced Icelanders and according to data from the 1,000 Genome Project. However, it has 33 variants that have high D ′ (above 0.86) and an r 2 between 0.2 and 0.5 ( Supplementary Table S2 ). Essentially, this means that other variants (mutations) cannot be identified in our data set, which can fully account for the observed association signal reported here. Bioinformatic analysis of RCC risk variant We cross referenced the location of rs35252396 against potential biological functional features according to the Encyclopedia of DNA Elements project [13] . rs35252396 is located within a predicted DNaseI hotspot shown to have a strong signal strength in three renal cell lines (RPTEC, HRE and HRCEpiC; Supplementary Fig. S1 and Supplementary Table S3 ). We also noted, based on a FAIRE-Seq analysis (Formaldehyde-Assisted Isolation of Regulatory Element), that rs35252396 is located at a reported regulatory site in the renal cell adenocarcinoma cell line RCC_7860. This site has also been shown to bind KAP1 and ZNF263 transcription factors, according to a ChIP-Seq analysis, in the embryonic kidney cell lines HEK293 and HEK293-T-Rex, respectively. Furthermore, rs35252396 is located within a chromatin interaction site, predicted to interact with the 5′-untranslated region of MYC based on a ChIA-PET assay analysis of the leukemia cell line k562 ( Supplementary Fig. S1 and Supplementary Table S4 ). Finally, the Ensembl Genome Browser defined rs35252396 as a regulatory region variant with a biological function in several different cell lines. Whether any of these observations sheds light on the association with RCC remains to be shown. In summary, we have discovered a new RCC risk variant at the 8q24 locus, a locus shown to be associated with cancers in several organs but not previously with kidney cancer. Interestingly, this variant has no strongly correlated variants and it is located within several potential regulatory regions of the genome. Otherwise, the risk profile of this new variant is comparable to other GWAS-based discovered risk variants in being common and conferring moderate risk of the disease. However, the discovery of each new RCC risk variant may ultimately contribute to earlier detection and better treatment of the disease. Study populations The Icelandic study population is based on a nationwide list from the ICR containing 1,651 Icelandic RCC patients diagnosed from 1 January 1955, to 31 December 2011. The Icelandic RCC sample collection included 575 patients who were recruited from November 2000 until June 2012. A total of 1,505 patients were included in the current study, of which 575 had genotypes from a genome-wide SNP genotyping effort, using the Infinium II assay method and the Sentrix HumanHap300 BeadChip (Illumina, San Diego, CA, USA), and 930 had imputed genotypes based on genotypic information from first- or second-degree relatives who have been chip genotyped. In total, ~10% of the RCC patients had carcinomas of the papillary, chromophobe-mixed or unknown histological subtypes. Of the 1,505 RCC patients, 14 were among the 2,230 individuals who had been whole-genome sequenced. The mean age at diagnosis was 66 years for RCC patients in our study. The 67,725 control individuals (25,875 had variants imputed based on chip genotypes and 41,850 had variants imputed with family-based methods) comprises individuals recruited through different genetic research projects at deCODE. The controls have been diagnosed with common diseases of the cardiovascular system (for example, stroke or myocardial infraction), psychiatric and neurological diseases (for example, schizophrenia and bipolar disorder), endocrine and autoimmune system (for example, type 2 diabetes and asthma), malignant diseases other than RCC and individuals randomly selected from the Icelandic genealogical database. The controls had a mean age of 84 years and the range was from 8 to 105 years. The controls were absent from the nationwide list of RCC patients according to the ICR. The study was approved by the Data Protection Commission of Iceland and the National Bioethics Committee of Iceland. Written informed consent was obtained from all patients and controls. Personal identifiers associated with medical information and blood samples were encrypted with a third-party encryption system as previously described [14] . The Dutch RCC sample series ( N =776) consist of a population-based series ( N =427) and a hospital-based series ( N =349). The hospital-based series has been described in a previous publication [15] . Patients with urological diseases were recruited through the outpatient urology clinic of the Radboud University Medical Center (RUMC) from January 1999 onwards. The ~10,000 patients who participated in this study gave informed consent for the study and for linking their data with disease registries. The study was linked with the Dutch population-based cancer registry to identify patients who were diagnosed with renal cell cancer. Three hundred and forty-nine patients were identified. The (non-overlapping) population-based series has been recruited in 2009. Patients were identified through the population-based regional cancer registry held by the Comprehensive Cancer Centre East, Nijmegen. Patients diagnosed between 1995 and 2008, <75 years of age, were selected, and their vital status and current addresses updated through the hospital information systems of the seven community hospitals and one university hospital (RUMC) that are covered by the cancer registry. All patients still alive on 1 February 2009 were invited to the study by the Comprehensive Cancer Center on behalf of the patients’ treating physicians. In case of consent, patients were sent a lifestyle questionnaire to fill out, and blood samples were collected by Thrombosis Service centers that hold offices in all the communities in the region. Seven hundred and eight patients were invited to participate; 465 responded positively, and data and samples were collected from 427 patients. All the patients who were selected for analyses are of self-reported European descent. Clinical data were obtained through the cancer registry. The study protocol was approved by the Institutional Review Board of the Radboud University Medical Centre (RUMC) and all study subjects gave written informed consent. The Dutch controls were recruited within a project entitled ‘Nijmegen Biomedical Study’ (NBS). The details of this study were reported previously [16] . Briefly, this is a population-based survey conducted by the Department for Health Evidence and the Department of Clinical Chemistry of the RUMC, in which 9,371 individuals participated from a total of 22,500 age- and sex-stratified invitees, randomly selected from the general population of the municipality of Nijmegen. Control individuals from the NBS were invited to participate in a study on gene–environment interactions in multifactorial diseases, such as cancer. The 2,366 controls are a subsample of all the participants to the NBS and were cancer free at the date of recruitment. All control subjects were fully informed about the goals and the procedures of the study, and signed an informed consent form. The study protocols of the NBS were approved by the Institutional Review Board of the RUMC. The Spanish study population used in this study consisted of 130 pathologically confirmed RCC. The cases were recruited from the Oncology Department of Zaragoza Hospital in Zaragoza, Spain, from June 2004 to September 2009. Clinical information, including age at onset, grade and stage, was obtained from medical records. The average age at diagnosis for the patients was 63 years. The 1,406 Spanish control individuals were approached at the University Hospital in Zaragoza and were cancer free at the time of recruitment. All study subjects were of self-reported European descent and study protocols were approved by the Institutional Review Board of Zaragoza University Hospital. All subjects gave written informed consent. Illumina genome-wide genotyping The Icelandic chip-typed samples were assayed with the Illumina Human Hap300, Hap CNV370, Hap 610, 1M or Omni-1 Quad bead chips at deCODE genetics. SNPs were excluded if they had yield <95%, minor allele frequency <1% in the population or significant deviation from the Hardy–Weinberg equilibrium in the controls ( P <0.001), if they produced an excessive inheritance error rate (>0.001), or if there was substantial difference in allele frequency between chip types (from just a single chip if that resolved all differences, but from all chips otherwise). All samples with a call rate <97% were excluded from the analysis. The final set of SNPs used for long-range phasing composed of 785,863 SNPs. We note that rs35252396(CG/AC) has also been annotated as two consecutive single-nucleotide variations, rs6470588(A/C) and rs6470589(C/G). rs6470588 is present on the Illumina chips used to genotype the Icelandic sample. Single-track assay SNP genotyping and Sanger sequencing Genotyping of rs35252396 as reported in Table 2 for patients and controls from the Netherlands and Spain was carried out by deCODE genetics in Reykjavik, Iceland, applying the Centaurus [17] (Nanogen) single-track assay platform. To validate the imputed Icelandic association results for rs35252396, we directly genotyped 1,678 Icelandic study subjects using a single-track assay. The correlation ( r ) between the two genotyping methods was 0.98. For confirming the genotypes from the single-track assay, we Sanger sequenced 395 individuals from Iceland, the Netherlands and Spain. The correlation between these two data sets was high ( r =0.97). Whole-genome sequencing and SNP genotype calling Of the 2,230 individuals whole-genome sequenced and used in the current study, 14 have been diagnosed with RCC according to the nationwide list maintained by the ICR. Paired-end libraries for sequencing were prepared according to the manufacturer’s instructions (Illumina). In short, ~5 μg of genomic DNA, isolated from frozen blood samples, were fragmented to a mean target size of 300 bp using a Covaris E210 instrument. The resulting fragmented DNA was end repaired using T4 and Klenow polymerases, and T4 polynucleotide kinase with 10 mM dNTP, followed by the addition of an ‘A’ base at the ends using Klenow exo fragment (3′ to 5′-exo minus) and dATP (1 mM). Sequencing adaptors containing ‘T’ overhangs were ligated to the DNA products followed by agarose (2%) gel electrophoresis. Fragments of about 400 bp were isolated from the gels (QIAGEN Gel Extraction Kit), and the adaptor-modified DNA fragments were PCR enriched for ten cycles using Phusion DNA polymerase (Finnzymes Oy) and PCR primers PE 1.0 and PE 2.0 (Illumina). Enriched libraries were further purified using agarose (2%) gel electrophoresis as described above. The quality and concentration of the libraries were assessed with the Agilent 2100 Bioanalyzer using the DNA 1000 LabChip (Agilent). Barcoded libraries were stored at −20 °C. All steps in the workflow were monitored using an in-house laboratory information management system with barcode tracking of all samples and reagents. Template DNA fragments were hybridized to the surface of flow cells (Illumina PE flowcell, v4) and amplified to form clusters using the Illumina cBot. In brief, DNA (3–10 pM) was denatured, followed by hybridization to grafted adaptors on the flowcell. Isothermal bridge amplification using Phusion polymerase was then followed by linearization of the bridged DNA, denaturation, blocking of 3′-ends and hybridization of the sequencing primer. Sequencing by synthesis was performed on Illumina GAIIx instruments equipped with paired-end modules. Paired-end libraries for whole-genome sequencing were sequenced using either 2 × 101 or 2 × 120 cycles of incorporation and imaging with Illumina sequencing kits, v4 or v5 (TruSeq). Each library or sample was initially run on a single lane for validation, followed by further sequencing of ≥4 lanes with targeted raw cluster densities of 500–700 k mm −2 , depending on the version of the data imaging and analysis packages. Imaging and analysis of the data was performed using SCS2.6 /RTA1.6, SCS2.8/RTA1.8 or SCS2.9&RTA1.9 software packages from Illumina, respectively. Real-time analysis involved conversion of image data to base calling in real time. Reads were aligned to NCBI Build 36 of the human reference sequence using Burrows-Wheeler Aligner 0.5.9 (ref. 18 ). Alignments were merged into a single BAM file and marked for duplicates using Picard 1.55 ( http://picard.sourceforge.net/ ). Only non-duplicate reads were used for the downstream analyses. Variants were called using Genome Analysis Toolkit, (GenomeAnalysisTK) 1.2-29-g0acaf2d (ref. 19 ), by applying base quality score recalibration, INDEL realignment and performing SNP and INDEL discovery and genotyping using standard hard filtering [20] . Variants were annotated using SNPeff and Genome Analysis Toolkit 1.4-9-g1f1233b with only the highest-impact effect [19] . The allele frequency used for filtering was based on phased genotypes of 38.5 million SNPs and INDELs from the 2,230 whole-genome-sequenced Icelanders. Long-range phasing and genotype imputation Long-range phasing of all chip-genotyped individuals was performed with methods described previously [8] , [21] , [22] , [23] , [24] . In brief, phasing is achieved using an iterative algorithm, which phases a single proband at a time given the available phasing information about everyone else that shares a long haplotype identically by state with the proband. Given the large fraction of the Icelandic population that has been chip typed, accurate long-range phasing is available genome wide for all chip-typed Icelanders. We imputed the SNPs identified and genotyped through sequencing the whole genomes of 2,230 Icelanders into the additional 92,855 Icelanders who had been chip typed and phased with long-range phasing. These imputations are performed based on long haplotype sharing based on the chip SNPs and were performed using the same model as used by IMPUTE [25] . The genotype data from sequencing can be ambiguous owing to low sequencing coverage. To phase the sequencing genotypes, an iterative algorithm was applied for each SNP with alleles 0 and 1. We let H be the long-range-phased haplotypes of the sequenced individuals and applied the following algorithm: For each haplotype h in H , use the hidden Markov model (HMM) of IMPUTE to calculate for every other k in H , γ h,k , (see details for calculating γ h,k below). For every h in H , initialize the parameter θ h , which specifies how likely the one allele of the SNP is to occur on the background of h from the genotype likelihoods obtained from sequencing. The genotype likelihood L g is the probability of the observed sequencing data at the SNP for a given individual assuming g is the true genotype at the SNP. If L 0 , L 1 and L 2 are the likelihoods of the genotypes 0, 1 and 2 in the individual that carries h , then set : For every pair of haplotypes h and k in H that are carried by the same individual, use the other haplotypes in H to predict the genotype of the SNP on the backgrounds of h and k : and Combining these predictions with the genotype likelihoods from sequencing gives un-normalized updated phased genotype probabilities: and Now use these values to update θ h and θ k to: and Repeat step 3 when the maximum difference between iterations is greater than a convergence threshold ε . We used ε =10 −7 . Given the long-range-phased haplotypes and θ , the allele of the SNP on a new haplotype h not in H , is imputed as . The above algorithm can easily be extended to handle simple family structures such as parent–offspring pairs and triads by letting the P distribution run over all founder haplotypes in the family structure. The algorithm also extends trivially to the X chromosome. If source genotype data are only ambiguous in phase, such as chip genotype data, then the algorithm is still applied; however, all but one of the L s will be 0. In some instances, the reference set was intentionally enriched for carriers of the minor allele of a rare SNP to improve imputation accuracy. In this case, expected allele counts will be biased toward the minor allele of the SNP. Call the enrichment of the minor allele E and let θ ′ be the expected minor allele count calculated from the naive imputation method and let θ be the unbiased expected allele count, then: and hence, This adjustment was applied to all imputations based on enriched imputations sets. We note that if θ ′ is 0 or 1, then θ will also be 0 or 1, respectively. The coefficients γ h,k are calculated based on the same HMM model as that used by IMPUTE. Given a haplotype h in H , γ h,k are calculated simultaneously for all . Assuming that at each marker i the haplotype h has a common ancestor with a haplotype in and denote the variable indicating this with the latent variable , the hidden variable in the HMM, then Given the Markov assumtption of the HMM, the model is fully specified by emission and transition probabilities. We define the emission probabilities of the HMM at each marker i as: where λ can be thought of as a penalty for a mismatch. We used λ =10 −7 in our implementation. We define the transmission probabilities of the HMM model as: where N is the number of haplotypes in , which for autosomal chromosomes is 2(2,230−1) here, and , where r i is the genetic distance between markers i −1 and i according to the most recent version of the deCODE genetic map [24] and N e was originally meant to be an estimate of the effective number of haplotypes in the population that our sample comes from, we used N e =7,000. These definitions fully specify the probability distribution . Calculating γ h,k for a single haplotype requires O ( MN ) operations, where N is the number of haplotypes and M is the number of markers. As these calculations can be performed for one haplotype at a time, the calculations can be parallelized across a computer cluster for efficiency. In practice, most of the γ h,k will be close to zero and can be safely ignored (we used a threshold of 10 −6 of the largest value at each marker for each h ), greatly reducing storage requirements. These calculations took ~21 days on a cluster of 800 computing nodes. In addition to imputing sequence variants from the whole-genome sequencing effort into chip-genotyped individuals, we also performed a second imputation step where genotypes were imputed into relatives of chip-genotyped individuals. The inputs into the second imputation step are the fully phased (in particular, every allele has been assigned a parent of origin) imputed and chip-type genotypes of the available chip-typed individuals. The algorithm used to perform the second imputation step consists of the following steps. For each ungenotyped individual (the proband), find all chip-genotyped individuals within two meiosis of the individual. The six possible types of two meiosis relatives of the proband are (ignoring more complicated relationships due to pedigree loops) as follows: parents, full and half siblings, grandparents, children and grandchildren. If all pedigree paths from the proband to a genotyped relative go through other genotyped relatives, then that relative is excluded. For example, if a parent of the proband is genotyped, then the proband’s grandparents through that parent are excluded. If the number of meiosis in the pedigree around the proband exceeds a threshold (we used 12), then relatives are removed from the pedigree until the number of meiosis falls below 12, to reduce computational complexity. At every point in the genome, calculate the probability for each genotyped relative sharing with the proband based on the autosomal SNPs used for phasing. A multipoint algorithm based on the HMM Lander–Green multipoint linkage algorithm using fast Fourier transforms is used to calculate these sharing probabilities [26] , [27] . First, single point-sharing probabilities are calculated by dividing the genome into 0.5 cM bins and using the haplotypes over these bins as alleles. If there are n informative haplotypes in the pedigree around the proband, it is denoted by , the inheritance vector (sharing pattern) [26] . Haplotypes that are the same, except at most at a single SNP, are treated as identical. Given the haplotype frequencies in each bin, the single point distribution, , can be calculated as in classical multipoint linkage analysis [26] . When the haplotypes in the pedigree are incompatible over a bin, then a uniform probability distribution was used for that bin, The most common causes for such incompatibilities are recombination in members belonging to the pedigree, phasing errors and genotyping errors. Note that as the input genotypes are fully phased, the single point information is substantially more informative than for unphased genotyped, in particular one haplotype of the parent of a genotyped child is always known. The single point distributions are then convolved using the multipoint algorithm to obtain multipoint sharing probabilities at the centre of each bin just as in the original Lander–Green algorithm [26] . Genetic distances were obtained from the most recent version of the deCODE genetic map [24] . On the sharing probabilities at the centre of each bin, all the SNPs from the whole-genome sequencing are imputed into the proband. We now show how to impute the genotype of the paternal allele of a SNP located at x , flanked by bins with centers at x left and x right . Starting with the left bin, going through all possible inheritance vectors v , let I v be the set of haplotypes of genotyped individuals that share identically by descent within the pedigree with the proband’s paternal haplotype given the inheritance vector v and P ( v ) be the probability of v at the left bin—this is the output from step 2 above—and let e i be the expected allele count of the SNP for haplotype i . Then, is the expected allele count of the paternal haplotype of the proband, given v , and an overall estimate of the allele count, given the sharing distribution at the left bin, is obtained from: If I v is empty, then no relative shares with the proband’s paternal haplotype given v , and thus there is no information about the allele count. We therefore store the probability that some genotyped relative shared the proband’s paternal haplotype, and an expected allele count, conditional on the proband’s paternal haplotype being shared by at least one genotyped relative: In the same way, we calculated O right and c right . Linear interpolation is then used to get an estimates at the SNP from the two flanking bins: If is an estimate of the population frequency of the SNP then is an estimate of the allele count for the proband’s paternal haplotype. Similarly, an expected allele count can be obtained for the proband’s maternal haplotype. The informativeness of genotype imputation was estimated by the ratio of the variance of imputed expected allele counts and the variance of the actual allele counts: where is the allele count. was estimated by the observed variance of the imputed expected counts and was estimated by p (1− p ), where p is the allele frequency. For the present study, when imputed genotypes are used, the information value for all SNPs is >0.90. The imputed genotype information measure value for rs35252396 is 0.99. Case–control association testing Logistic regression was used to test for association between SNPs and disease, treating disease status as the response and expected genotype counts from imputation or allele counts from direct genotyping as covariates. Testing was performed using the likelihood ratio statistic. When testing for association based on the imputed genotypes, controls were matched to cases based on the informativeness of the imputed genotypes, such that for each case C controls of matching informativeness where chosen. Failing to match cases and controls will lead to a highly inflated genomic control factor, and in some cases may lead to spurious false-positive findings. The informativeness of each of the imputation of each one of an individual’s haplotypes was estimated by taking the average of over all SNPs imputed for the individual, where e is the expected allele count for the haplotype at the SNP and is the population frequency of the SNP. This measure has the property that it is 0 if the population frequency is imputed, , and 1 if either allele is imputed with full certainty, . The mean informativeness values cluster into groups corresponding to the most common pedigree configurations used in the imputation, such as imputing from parent into child or from child into parent. On the basis of this clustering of imputation informativeness, we divided the haplotypes of individuals into 7 groups of varying informativeness, which created 27 groups of individuals of similar imputation informativeness, 7 groups of individuals with both haplotypes having similar informativeness, 21 groups of individuals with the 2 haplotypes having different informativeness, minus the 1 group of individuals with neither haplotype being imputed well. Within each group, we calculate the ratio of the number of controls and the number of cases, and choose the largest integer C that was less than this ratio in all the groups. For example, if in one group there are 10.3 times as many controls as cases and if in all other groups this ratio was greater, then we would set C =10 and, within each group, randomly select ten times as many controls as there are cases. For the RCC study, we used C =45. Inflation factor adjustment To account for the relatedness and stratification within our case and control sample sets, we applied the method of genomic control based on chip markers ( Fig. 1 ). For the RCC GWAS, the correction factor based on genomic control is 1.26. Genomic annotation analysis We carried out a search for overlaps between the location of rs35252396 and predicted biological features. We retrieved data from UCSC test browser (HG19 build 37) [28] , and inspected manually all feature tracks relevant to kidney tissue and identified those features that overlapped with the location of the variant. These are recognized draft quality data and were used as reported without quality filtering. How to cite this article: Gudmundsson, J. et al. A common variant at 8q24.21 is associated with renal cell cancer. Nat. Commun. 4:2776 doi: 10.1038/ncomms3776 (2013).